Flocking at a distance in active granular matter The self-organized motion of vast numbers of creatures in a single direction is a spectacular example of emergent order. Here, we recreate this phenomenon using actuated nonliving components. We report here that millimetre-sized tapered rods, rendered motile by contact with an underlying vibrated surface and interacting through a medium of spherical beads, undergo a phase transition to a state of spontaneous alignment of velocities and orientations above a threshold bead area fraction. Guided by a detailed simulation model, we construct an analytical theory of this flocking transition, with two ingredients: a moving rod drags beads; neighbouring rods reorient in the resulting flow like a weathercock in the wind. Theory and experiment agree on the structure of our phase diagram in the plane of rod and bead concentrations and power-law spatial correlations near the phase boundary. Our discovery suggests possible new mechanisms for the collective transport of particulate or cellular matter. The flocking of animals [1] , [2] , [3] , [4] relies on organisms sensing each other’s presence, orientation and direction of movement. Physical scientists interested in this spontaneous breaking of rotation invariance in living systems have adopted a variety of approaches to the problem [5] , [6] , [7] , including experiments in vivo and in vitro [8] , computer simulations and theory. Artificial analogues of self-propulsion [9] , [10] , [11] , [12] , [13] , [14] , [15] , [16] are currently a subject of intense interest, both as a controlled testing ground for theoretical predictions and as a rich source of new phenomena and applications. We focus here on the case of macroscopic particles with a stepwise tapered rod-like shape, with inelasticity and static friction, placed on a rapidly vibrating surface. The tilt of the particle takes up the vibrational energy and, through a frictional mechanism already described elsewhere [9] , [17] , [18] , [19] , transduces it into directed motion along the surface. It is proper to regard such particles as self-propelling: the sustained energy input from the vibrating surface is nutrient or fuel, the tilt of the particle is the motor coordinate, the direction of motion is set by the particle orientation and not by an external force and the net in-plane force on particle plus base is zero. The motility mechanism can be viewed as a noisy ratchet [20] with the novelty that the asymmetry is carried not by the substrate but by the particle, as in ref. 21 . A single such motile rod on a bare vibrated surface translates, with mean speed 0.36 cm s −1 and standard deviation 0.25 cm s −1 , where the statistics is obtained from 150 rods, primarily in the direction of the vector from its thick end to its thin end. That vector itself executes rotational diffusion, losing memory of its initial orientation on long enough timescales. As a result, the centre of mass of the rod describes a persistent two-dimensional random walk in the plane of the surface on which it lies. Anisotropy is crucial: spheres, lacking a distinguished axis, cannot tilt and thus cannot achieve motility, that is, self-propulsion, by means of the mechanism that animates the rods. A sphere can move laterally only if pushed or dragged by the motile rods; an isolated sphere on a vibrating surface simply bounces in place [18] , [19] . The movements of a single motile rod amidst a sea of spherical beads were shown earlier [18] to display some remarkable statistical properties as a consequence of the obstacles to rod motion presented by the beads. In the present work we look for novel interaction effects, structural or dynamical in origin, in the collective behaviour of motile rods dispersed among spherical beads. Our curiosity is amply rewarded: we find that the rods self-organize into a globally oriented moving state at a remarkably low concentration provided the bead background is dense enough. A well-defined phase transition separates this ordered state or flock from the disordered isotropic phase. We create a detailed mechanistic simulation model of this system, which reproduces the phenomena observed and uncovers the underlying physical processes. We integrate the insights from experiment and simulation into a simple analytical theory whose predictions are borne out by our observations. Our work demonstrates for the first time the formation of a true flock in a collection of dry grains. Our discovery that a small concentration of motile particles can coherently transport a large passive cargo, with an efficiency that increases with the load, could find applications in granular flow. We speculate further that the mutual interaction of a small population of motile living organisms and a background of non-motile material could yield self-organization of the former and enhanced transport of the latter. 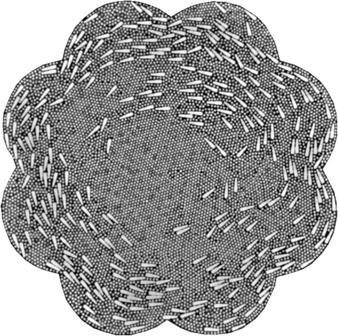Figure 1: A granular flock. A monolayer of millimetre-sized tapered brass rods align spontaneously on a vibrating surface amidst a background of aluminium beads. Bead and rod area fractions are 0.51 and 0.16 respectively. Experimental results Figure 1 shows a representative image of our granular flock. Despite their low concentration the rods display a high degree of orientational order. This and further results emerge from our experiments on a mixture of stepwise tapered rods and spherical beads confined between surfaces subjected to rapid vertical vibration (see Fig. 2a and Methods). The system is initialized by introducing the beads into the sample cell and distributing the rods amidst the beads, to yield a homogeneous rod–bead monolayer. We then study the nature of the statistically stationary state of the vibrated rod–bead mixture as a function of the area fractions Φ b and Φ r , defined as the fraction of the surface covered by the two-dimensional projections of the beads and rods, respectively. We monitor the centroid positions r i of all the particles and the tail-to-head unit vectors n i , where i labels the particle in question, and all vectors lie in the horizontal plane. Figure 1: A granular flock. A monolayer of millimetre-sized tapered brass rods align spontaneously on a vibrating surface amidst a background of aluminium beads. Bead and rod area fractions are 0.51 and 0.16 respectively. 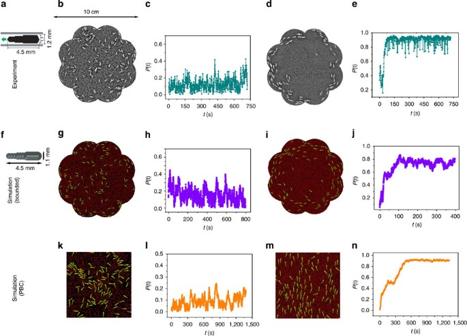Figure 2: Structure and kinetics of the disordered and ordered states. (a) Dimensions and confinement geometry of the polar rod used in the experiment, with arrow indicating direction of self-propulsion. (b–e) Typical configuration and corresponding time-evolution of polar order parameter in the disordered phase, bead and rod area fractionsΦb=0.41,Φr=0.05 (b,c), and in the ordered phase,Φb=0.68,Φr=0.05 (d,e); for the simulation in the flower geometry: (f) rod used in simulation, (g–j) as in (b–e):Φb=0.48,Φr=0.06 (g,h),Φb=0.66,Φr=0.06 (i,j); for the simulation with periodic boundary conditions, configuration and order-parameter evolution for the disordered phase,Φb=0.20,Φr=0.11 (k,l) and the ordered phase,Φb=0.60,Φr=0.11 (m,n). Full size image Figure 2: Structure and kinetics of the disordered and ordered states. ( a ) Dimensions and confinement geometry of the polar rod used in the experiment, with arrow indicating direction of self-propulsion. ( b – e ) Typical configuration and corresponding time-evolution of polar order parameter in the disordered phase, bead and rod area fractions Φ b =0.41, Φ r =0.05 ( b , c ), and in the ordered phase, Φ b =0.68, Φ r =0.05 ( d , e ); for the simulation in the flower geometry: ( f ) rod used in simulation, ( g – j ) as in ( b – e ): Φ b =0.48, Φ r =0.06 ( g , h ), Φ b =0.66, Φ r =0.06 ( i , j ); for the simulation with periodic boundary conditions, configuration and order-parameter evolution for the disordered phase, Φ b =0.20, Φ r =0.11 ( k , l ) and the ordered phase, Φ b =0.60, Φ r =0.11 ( m , n ). Full size image With increasing Φ b (or, less surprisingly, Φ r ) the system is seen to undergo a phase transition from a disordered state to one in which the rod orientation vectors are aligned. Correspondingly, the rods move in random directions in the low-density state ( Fig. 2b and Supplementary Movie 1 ) and coherently at high densities ( Fig. 2d and Supplementary Movie 2 ). At long times the global movement in the ordered phase is a clockwise or anticlockwise circulation with equal probability ( Supplementary Fig. 1 ), with the orientation vectors aligned parallel to the boundary. The direction of circulation once selected does not change for the duration of the experiment. We have checked that neither crystalline order nor mechanical rigidity of the bead bed is an essential ingredient in promoting the flocking of the rods. For example, the flock in Fig. 1 is on a liquid-like bead background. Further, rods in an amorphous bead bed, generated by using a mixture of bead sizes, are also seen to self-organize into a flock ( Supplementary Fig. 2 and Supplementary Note 1 ). Creating and maintaining a homogeneous state in bidisperse systems is complicated by size-segregation effects, which is why we have continued to work with beads of a single size. The rich physics that enters when the bead medium is a single- or multidomain crystal requires a separate study, now underway. In a confined geometry the simplest flock consists of particles globally circulating around a common centre, which is the motion seen in our experiments. Accordingly, we resolve n i into local polar-coordinate components , which we use to evaluate the order parameter P ≡‹ p i › distinguishing isotropic and oriented states, and G ( r )=‹ p i · p j › r − P 2 , which measures correlations of orientational fluctuations about the mean for pairs i , j of rods with separation | r i − r j |= r . The instantaneous in-plane bead-velocity unit vectors u i , transformed to the local polar frame to give , provide another measure of flocking, v ≡‹ v i ›. The averaging denoted by the angle brackets is carried out over all rods and over all times in the steady state for P , about 100 statistically independent images for G ( r ) and 25 frames for v (frame rate=40 s −1 , and the plate is vibrated at 200 Hz). The disordered and ordered phases are most clearly distinguished by growth kinetics. Figure 2c shows a typical disordered state with the magnitude P(t) ≡| P ( t )| of the instantaneous order parameter, averaged over rods but not over time t , fluctuating just above zero, and Fig. 2e presents an ordered state where P ( t ) grows and saturates to a value close to 1, which implies that polar rods are now moving parallel to the boundary. We construct a phase diagram based on the steady-state value of P as shown in Fig. 3a . For Φ r >0.025 we find that P increases abruptly across the line Φ b + kΦ r ≃ 0.65, k ≃ 2. We identify this line, provisionally, as the location of the nonequilibrium phase transition between the disordered and ordered states, bearing in mind the effects of finite size and the sample boundary. Correspondingly, Fig. 3c shows the experimentally measured polar order parameter as a function of Φ b for Φ r =0.08. At the smallest values of Φ r the phase boundary bends sharply upwards, possibly implying a true lower limit to the Φ r required to produce a flock regardless of Φ b . At the highest densities arrested states are observed, where rods either jam against the particles of the bead medium or cluster along the boundary ( Supplementary Fig. 3a ). 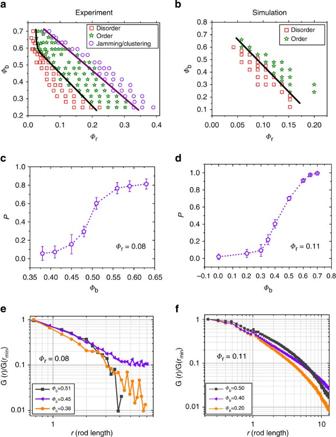Figure 3: Flocking phase transition and growth of correlations. (a) Experimental phase diagram in theΦb−Φrplane, showing the phase boundary between the isotropic phase and the flock. Clustering at the sample boundary sets in at high concentration. (b) Simulation phase diagram in the flower geometry reproduces the flocking transition. We have not explored concentrations at which boundary clustering is expected. Increase in polar order parameterPas function ofΦbfor experiments (c) and simulations (d). The error bars correspond to the standard deviation ofP. Orientational correlation function from experiments (e) and simulations in a 55.1-rod-length periodic box (f) at variousΦbat a fixedΦr. A considerable range of power-law correlations is seen asΦbincreases. Figure 3e reports the variation of the steady-state orientational correlations G ( r ) (scaled by its value at the smallest r ) of the rods as the system approaches and then crosses the phase boundary. For Φ b =0.45, spatial correlations consistent with a power-law are seen, while for larger or smaller Φ b , safely within the ordered or the disordered phase, correlations decay more rapidly. These observations can consistently be interpreted as pretransitional fluctuations in the vicinity of a nonequilibrium phase transition, although the system sizes explored are too small to permit a claim about the order of the transition. As effects of finite size limit the accuracy of our estimates of the value of the order parameter and the location of the phase transition, we present in Supplementary Fig. 4a the correlation functions of the orientation without the mean subtracted. The flocking of the polar rods is accompanied by coherent motion of the beads ( Fig. 4a ) as well, as measured by the bead-velocity order parameter v , which shows the same growth kinetics as P ( Fig. 4b ). Figure 3: Flocking phase transition and growth of correlations. ( a ) Experimental phase diagram in the Φ b − Φ r plane, showing the phase boundary between the isotropic phase and the flock. Clustering at the sample boundary sets in at high concentration. ( b ) Simulation phase diagram in the flower geometry reproduces the flocking transition. We have not explored concentrations at which boundary clustering is expected. Increase in polar order parameter P as function of Φ b for experiments ( c ) and simulations ( d ). The error bars correspond to the standard deviation of P . Orientational correlation function from experiments ( e ) and simulations in a 55.1-rod-length periodic box ( f ) at various Φ b at a fixed Φ r . A considerable range of power-law correlations is seen as Φ b increases. 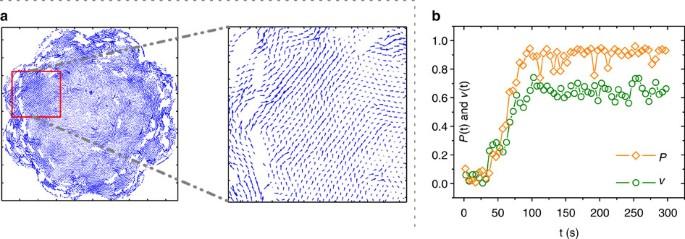Figure 4: Correlation between the dynamics of the polar rods and the bead medium. (a) Arrows in the zoom show the coherent velocity field of the bead medium in the ordered phase withΦb=0.66 andΦr=0.06. Blank regions are occupied by polar rods. (b) The ordering kinetics of the bead velocity field tracks that of the polar orientation. Full size image Figure 4: Correlation between the dynamics of the polar rods and the bead medium. ( a ) Arrows in the zoom show the coherent velocity field of the bead medium in the ordered phase with Φ b =0.66 and Φ r =0.06. Blank regions are occupied by polar rods. ( b ) The ordering kinetics of the bead velocity field tracks that of the polar orientation. Full size image Simulation results To understand the physics underlying this novel realization of a flocking transition, and to explore which of the many possible control parameters are essential, we create a computer model of tapered rods and spherical beads. For convenience in simulation the rods are constructed by joining overlapping spheres in a straight line ( Fig. 2f ), but their shape is chosen to resemble as closely as possible the stepwise tapered rods in the experiment. We have also tried other shapes such as a uniform taper and find qualitatively similar results which we do not present here. We carry out two types of studies, one in an enclosure constructed to imitate the experimental geometry, the other with periodic boundary conditions in the horizontal plane. In both cases the simulations, like the experiments, are three-dimensional, with a base and a lid permitting tightly confined motion in the third dimension. The energy input, precisely as in the experiment, is through vertical agitation of the container. The particles move according to the laws of Newtonian mechanics. Collisions of the particles with each other and with the bounding surfaces are governed by inelasticity and static Coulomb friction. We add a small rotational noise to the dynamics of individual rods. This improves the fidelity of our imitation of the experimental system, in which minute imperfections in particle shape and base or lid topography endow each rod with rotational diffusion even when no beads or other rods are present. Our simulation results can be seen in Figs 2g–j,k–n . In the ‘flower’ geometry we find precisely the behaviour seen in the experiment. Random motion at low area fraction ( Supplementary Movie 3 ) gives way to an ordered, circulating flock at high area fraction ( Supplementary Movie 4 ), and a phase diagram broadly corresponding to that in the experiment is obtained. The numerical experiment, moreover, can be performed in a periodic simulation box, eliminating the effects of sample boundaries. Figure 2k,l ( Supplementary Movie 5 ) and Fig. 2m,n ( Supplementary Movie 6 ) show that the order parameter, now measured in a global Cartesian frame, remains at values consistent with zero for all times at low Φ b , while at high Φ b it grows to saturation. Clear evidence of a flocking transition around Φ b ≃ 0.35 is seen in Fig. 3d showing polar order parameter as a function of bead area fraction. Consistent with these findings and with the experiments, Fig. 3f shows evidence of power-law correlations for Φ b =0.4, but appreciable curvature on a log–log plot for Φ b well in the ordered or the disordered regime. Increasing Φ b serves to promote orientational correlations for Φ r as low as 0.03 ( Supplementary Fig. 5 ). As in the experiments, we present the ‘unsubtracted’ correlation functions in Supplementary Fig. 4b . For good measure, we also investigate and rule out, in Supplementary Fig. 6 (and Supplementary Note 2 ), the possibility that the only role played by the beads is to reduce the rotational diffusion of rods. These simulation results establish beyond reasonable doubt that the phenomenon we observe is a phase transition, with the beads playing a direct role in mediating an aligning interaction among the rods. Finally, on theoretical grounds, in particular because the suspending medium of beads is compressible [16] , we expect large number fluctuations in our system as in standard flocking models of the Toner-Tu type [2] . In such systems, large-scale correlated particle currents arise as a result of the coupling to easily excited and slowly decaying variations in the orientation field, both in the ordered phase [2] and in the isotropic phase near onset [22] . In Methods we show that the separate conservation of rods and beads leaves unaltered the arguments [2] for anomalously large number fluctuations. We have carried out a limited set of numerical studies of fluctuations in the number density of rods in the ordered and disordered phases, and find an excess in both cases ( Fig. 5 ). Our simulation measurements of the standard deviation Δ N in the number of polar rods in regions containing ‹ N › particles on average show that grows with ‹ N ›. However, more extensive simulations or experiments are required for a useful fit to a power law or other dependence on ‹ N ›, and to probe the relation of this phenomenon to known sources [2] , [5] , [22] , [23] , [24] of enhanced density fluctuations in active systems. 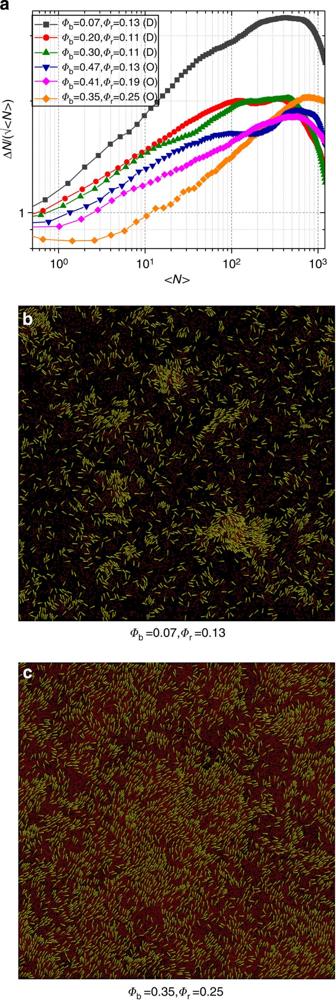Figure 5: Enhanced density fluctuations. (a) The scaled standard deviationin the number of polar rods, for regions containing ‹N› rods on average, is seen to grown with ‹N› for area fractions in the ordered (labelled O) and disordered (D) phases. (b) and (c) Representative images from the two phases. Figure 5: Enhanced density fluctuations. ( a ) The scaled standard deviation in the number of polar rods, for regions containing ‹ N › rods on average, is seen to grown with ‹ N › for area fractions in the ordered (labelled O) and disordered (D) phases. ( b ) and ( c ) Representative images from the two phases. Full size image Theory We now integrate the insights gained from experiment and simulation to construct a theory. The sequence of events in Fig. 6 also seen in simulation studies, shows that coherently moving polar rods are able to entrain a stray rod initially moving in the opposite direction, through the bead flow they generate, as seen in Supplementary Movies 2, 4 and 6 . These observations suggest that the coupling of flow and orientation lies at the heart of the phenomenon of flocking at a distance, as we now show through a minimal, universal hydrodynamic theory whose parameters and their dependence on Φ b are measured in our simulation. We also discuss the connection to the particular case of Bricard et al . 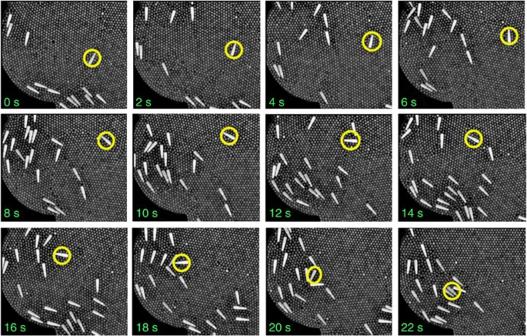Figure 6: Flowing beads reorient polar rods. A series of experimental images showing a stray polar rod brought into alignment with the rest of the flock as a consequence of bead flow. [16] Figure 6: Flowing beads reorient polar rods. A series of experimental images showing a stray polar rod brought into alignment with the rest of the flock as a consequence of bead flow. Full size image As we are concerned with large-scale ordering, we work with coarse-grained fields. Our system is a suspension of polar rods in a compressible two-dimensional fluid of beads on a substrate. The variables of interest are therefore the local order parameter P ( r , t ), given by the average of the orientation vectors p i of the polar rods, and the number densities ρ and σ of beads and rods, respectively, in a small neighbourhood around point r at time t . Below, for simplicity, we consider the limit of small rod concentration, and so treat only the bead density ρ ( r , t ). A treatment with both densities is in Methods. In addition, we include v ( r , t ), the average bead-velocity vector in the neighbourhood, as it has a crucial role in mediating the interactions that lead to order. In the dilute-rod limit v can be viewed as the total velocity field of both species. The equations of motion follow from a few general principles and some key elements of the dynamics of the system. Conservation of particles is embodied in the continuity equation Newton’s second law locally reads where we present only the leading-order terms in an expansion in powers of gradients and fields. In (2), Γ>0 damps motion with respect to the substrate and lid, the term in B can be viewed as describing pressure forces, driving flow downhill in density for B >0, and α measures the degree to which orientation of the polar rods gives rise to propulsive flow. We note in passing here that such a term was argued to arise [25] in the two-dimensional projection of the three-dimensional hydrodynamics of a suspension of motile organisms confined to a thin layer of fluid. We discuss below the somewhat different origin of the term in the case of our monolayer system. The viscosity η describes transmission of momentum in the plane of the system. The local order parameter P , again to leading order in gradients and fields, obeys where a measures the rate at which an initial polarization relaxes, presumably through rotational diffusion, and the magnitude and sign of A characterize the tendency of rods to orient parallel or antiparallel to concentration gradients [2] , [26] . The parameter λ determines the rate at which a uniform velocity (with respect to the confining walls) aligns the polarization. The parameter K governs spatial variations in the direction and magnitude of the order parameter. The ellipsis in (2) and (3) denotes contributions [2] at higher orders in p , v and ∇ , discussed in Methods. The terms with coefficients α and λ are the key players in (2) and (3). No symmetry rules out their existence; a phenomenological theory must therefore include them. However, the physics underlying these terms, especially as regards their signs, merits some discussion. Recall that p i for the i th rod points from the thick to the thin end. Depending on the detailed contact mechanics with the vibrating base, the rod could propel itself on average parallel or antiparallel to p i . Friction would cause the bead medium in the vicinity to be dragged in the direction of motion of the rod. A collection of such rods thus generates a force proportional to the mean polarization P . The parameter α measures the strength of this forcing. The magnitude of α should grow with the mean rod concentration and propulsion speed, and should further depend on the surface characteristics of a rod, which influence its ability to carry the ambient medium with it, by dragging or pushing. A rod with spontaneous motion parallel (antiparallel) to p i has α >0 ( α <0). By suitably engineering the geometry, mass distribution, surface properties and contact mechanics of a rod, and exploring a range of vibration parameters, it should be possible to make polar rods with a range of magnitudes and either sign of α ; the rods we work with here have α >0. The mechanics underlying λ is reminiscent of the interaction of wind with a weathercock. Imagine a single tapered rod lying athwart a uniform flow of particles over a surface. Although the momentum transfer is distributed uniformly across the rod, its mass is concentrated, and hence its pivot point shifted, towards one end. This leads to a net torque due to the flow, and a consequent rotation as shown in Fig. 7a . Geometrical arguments alone cannot determine the sign of λ and hence the sense of rotation, and self-propelling activity could influence its value. It should be possible to engineer λ <0 by using intrinsically higher-density material at the thin end, or a hollow interior at the thick end. 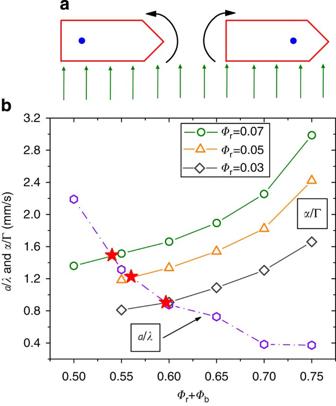Figure 7: Weathercock effect and location of the phase transition. (a) The direction in which the polar rod is rotated by a flow depends on its natural pivot point. (b)α/Γ is seen to grow anda/λto decrease with increasingΦb. Thus the flow velocity generated by a local polarization as well as the aligning power of bead flow grow with increasing bead concentration. The mean-field estimate of the flocking transition corresponds to the intersection of the two curves, marked by stars, whereāin Equation (4) changes sign from positive to negative asΦr+Φbis increased. Figure 7: Weathercock effect and location of the phase transition. ( a ) The direction in which the polar rod is rotated by a flow depends on its natural pivot point. ( b ) α /Γ is seen to grow and a / λ to decrease with increasing Φ b . Thus the flow velocity generated by a local polarization as well as the aligning power of bead flow grow with increasing bead concentration. The mean-field estimate of the flocking transition corresponds to the intersection of the two curves, marked by stars, where ā in Equation (4) changes sign from positive to negative as Φ r + Φ b is increased. Full size image The availability of a numerical simulation model provides independent measurements of all phenomenological parameters of importance to our theory. To measure λ , we place a single polar rod initially pointing in the x direction, and impose a flow of beads with velocity v in the y direction (see Supplementary Movie 7 ). By measuring the initial growth rate we estimate the parameter λ in (3), which we average over 50 such trials. Independently, by measuring the rotational relaxation of a single rod, we infer a . In a separate simulation, we impose a nonzero mean P by applying an orienting field on a collection of rods. Measuring the saturation value of the resulting macroscopic velocity yields α /Γ in (2). The damping Γ is readily estimated from the relaxation of an imposed initial velocity. Figure 7b shows the dependence of these key parameters on area fraction ρ 0 . We comment in Methods on the parameter A , which has only a minor role in our analysis. We ignore density variations in (3) and (2), replacing ρ by its mean value ρ 0 , which we treat as a parameter on which the coefficients depend. Working with the spatial Fourier components v q and P q of the velocity and order parameter at wavevector q , (2) then tells us that, on timescales long compared to ρ 0 /Γ, v q → α P q /(Γ+ ηq 2 ). Substituting this value for v in (3) we obtain, to order q 2 , where ā = a − λα /Γ and . The mechanism for spontaneous ordering now becomes clear. As λ is an increasing function of ρ 0 , ā can turn negative even if a is positive. The state P =0 is then linearly unstable, and a state with nonzero P on macroscopic scales will set in. Let us now test our theory using our simulation measurements of the parameters. First, for the proposed mechanism to work, ā must be less than a , that is, we predict λα /Γ>0. Our simulations show that a rod drags beads in the direction of its own motion and that the flow of beads rotates neighbouring rods to point in, and thus move in, the direction of the flow. Thus α and λ have the same sign, confirming the prediction. Second, Fig. 7b shows that as Φ r + Φ b is increased, α /Γ (for three values of Φ r ) increases and a / λ decreases, and the two quantities cross (that is, ā crosses zero) at a value of Φ r + Φ b , which decreases with increasing Φ r . Therefore the theory predicts a phase transition to an ordered phase with increasing area fraction, and negative slope to the phase boundary in the Φ r − Φ b plane, both of which are borne out by experiment. The intersection points in Fig. 7b , corresponding to the mean-field estimate of the threshold area fraction, are, not surprisingly, somewhat lower than the measured values in the simulation, Fig. 3b . Within our mean-field treatment ((4) or the parent equations (3) and (2)) it is straightforward to see that the transition has a continuous onset and a diverging correlation length . Our limited observations in experiment and simulation show an increasing correlation length upon approach to the transition. Experience with standard flocking models would suggest [27] instead a discontinuous transition, albeit with appreciable pretransitional fluctuations. Larger-scale simulation studies including finite-size scaling analyses, now in progress, will determine the character and spatial structure of the onset of order for our rod–bead flock. Note that orientability, motility and coupling to flow, rather than specifics of shape, were the essential ingredients of our theory. On symmetry grounds one cannot therefore rule out the possibility that the self-propelled disks of ref. 10 , in a background of non-motile particles, could flock through the mechanism reported here—provided flow can reorient the disks in the manner required. Our work is of importance as a remarkable example of cooperativity in active matter, with rods and beads giving rise to an order that the former could not achieve at such low concentration and the latter could not aspire to at all. It suggests an original mechanism for creating a coherent motile composite by introducing a small number of orientable motile particles into a medium containing non-motile components, that transmit motion more effectively as their concentration is increased. A static image of the ordered state would give no clue as to why the rods are lining up: the transmission of orientational information takes place through a viscous interaction which can be tuned through concentration. This works because our system is a monolayer, not a confined three-dimensional fluid. Momentum transfer in the vertical direction is governed by friction with the bounding base and lid. Only the transmission of momentum laterally in the plane of the system is governed by an effective viscosity arising from tangential forces between the beads with each other and with the rods. Our simulations show that in-plane viscous effects, as measured by α or η in (2), are enhanced by increasing bead concentration, while the out-of-plane damping Γ stays constant. It is this key feature that gives us a system in which the flocking tendency can be tuned by varying the concentration of the non-motile actors, the beads. Empirically, the system displays a flocking transition even if the bead medium is so concentrated that it crystallizes. Our simplified theory is restricted to the case where the system as a whole is fluid, not crystalline. How motile rods move through and transmit their motion and orientation through a highly ordered bead medium remains a major open problem. The hydrodynamic theory we have presented is indifferent to the precise origin of motility. It matters only that a polar, motile object drags ambient inert particles, whose flow in turn reorients neighbouring polar particles. There is a priori no reason why this cannot be realized in a system in which the motility mechanism does not require mechanical vibration or, for that matter, a vertical electric field as in ref. 16 . Could living matter take advantage of such a general mechanism? The reader should note that the flocking behaviour seen in our system was not inevitable, but relied on favourable signs of the parameters α (rods drag beads) and λ (the weathercock effect). An important direction that we are currently exploring is to design polar rods with the ‘wrong’ relative sign of α and λ . Indeed all the parameters α , Γ, λ and a can be manipulated at the scale of a single particle. Increasing rotational noise, perhaps by roughening particle surfaces or increasing the vibration amplitude, should increase a . Γ could be changed by roughening the base and lid. The tendency of a polar rod to point along the flow is quantified by λ . The shape and the mass distribution of the rod are the likely properties governing this parameter. It seems to us that there are two mechanisms behind the term α P in (2): dragging by tangential forces at the sides of a rod, and the pushing of beads at the head of a rod. A detailed exploration of the effects of shape and surface friction would allows us to manipulate α . Much remains to be explored about this granular flock. Deep in the ordered phase, the character of excitations about the uniform aligned state awaits study, as do the statistics of density and orientational fluctuations. Just past the apparent onset of order, does our system reproduce the banding instability of simple flocks, and is the character of this granular flocking phase transition discontinuous [27] ? What is the nature of the competition between kinetic arrest and flocking as concentrations are increased? Before closing, we return to the colloidal flock of Bricard et al . [16] , in which energy from a vertical electric field is transduced into rolling motion in a horizontal plane. In that system too, hydrodynamic coupling leads to a macroscopically aligned state of particle velocities. The most important distinguishing feature of our system is that the aligning interaction between the motile polar rods can be tuned by changing the concentration of the beads, which are themselves non-motile. Furthermore, the suspending medium, namely, the fluid of beads, is compressible (effects associated with overall incompressibility of grains plus air should arise in an airtight container. ), which rules out the suppression of fluctuations found by Bricard et al . [16] ; the rods carry an intrinsic shape polarity; the single-rod motility is not hydrodynamic in origin; the hydrodynamics at all scales in our monolayer system is that of a two-dimensional fluid on a dissipative substrate [28] ; the flow field around a single polar rod ( Supplementary Fig. 7 and Supplementary Note 3 ) is simply a screened monopole [29] . To summarize: we have created a system of macroscopic motile dry grains that flock spontaneously at low concentration, transmitting information about their orientation over large distances through the flow of an ambient medium of millimetre-sized beads. The beads, themselves non-motile, are cargo and coupling: increasing their number promotes flocking and enhances their own coherent transport. The simple and robust mechanism underlying this nonequilibrium phase transition prompts us to wonder about its possible wider relevance in living matter and industry. Experimental methods Our experiments are conducted on a mixture of macroscopic brass rods and aluminium beads. The rods [18] are 4.5 mm long, with diameter tapered in steps from 1.1 mm at the thick end or tail to 0.7 mm at the thin end or head, as shown in Fig. 2a . The beads are spheres of diameter 0.8 mm. The rod–bead mixture is confined to a monolayer in an experimental cell consisting of a shallow circular well in an aluminium plate whose dimensions and shape are shown in Fig. 2b . The plate is covered by a glass lid, and the distance w from plate to lid is 1.2 mm. The assembly is vibrated vertically by a magnetic shaker (LDS V406-PA100E). All our experiments are carried out at oscillation amplitude A =0.04 mm and frequency f =200 Hz, corresponding to a nondimensional shaking strength (2π f ) 2 A / g =7.0 where g is the acceleration due to gravity. The rods imitate self-propulsion by transducing the vertical vibration into fluctuating but persistent motion in the plane, in the tail-to-head direction [9] , [17] , [18] , [19] (the arrow in Fig. 2a ). We prevent accumulation of particles at the boundary, seen in Supplementary Fig. 2b , by the use of a flower-shaped sample cell [10] . Images of the collection of particles were acquired by high-speed camera (Basler acA2040-180 kc, 2,046 × 2,046 pixels giving a spatial resolution of 0.05 mm for our setup) at 40 frames per second and analysed in ImageJ ( http://rsb.info.nih.gov/ij/ ). Simulation methods Our simulation is time-driven, as particle shapes and the vibrating base and lid complicate the prediction of the next collision. All the interactions in the simulations are based on the impulse-based rigid body collision model [30] , [31] . Each tapered rod consists of equally spaced 13 overlapping spheres, seven of 1.1 mm diameter and three each of 0.88 and 0.72 mm ( Fig. 2f ), with mass density 8.7 g cm −3 corresponding to brass. The beads are represented by spheres of diameter 0.8 mm and mass density 2.7 g cm −3 of aluminium. The vertical positions of the vibrating base and lid at time t are A cos 2π ft + A and A cos 2π ft + A + w , respectively. All quantitative studies with periodic boundary conditions are all for a system size of 55.1 rod lengths; some videos use a different size. The rods in the experiment display rotational diffusion as a result of slight imperfections in the shape or substrate roughness. Lacking such asperities, our numerical rods need to be supplied with rotational noise: if a rod collides with the bed or the lid with relative velocity ε rel of contact points normal to contact plane, an extra angular velocity ω z = εε rel η is supplied to the rods. Here η =±1 with equal probability. The strength ε is a control parameter. To closely match the experimentally observed single-particle dynamics, we choose the friction and restitution coefficients μ and e to be 0.05 and 0.3 for particle–particle collisions, 0.01 and 0.3 for bead–wall (base, lid and lateral boundary) collisions, 0.03 and 0.1 for rod–base(or rod–lid) collisions, 0.01 and 0.3 for rod–boundary collisions, respectively. Between collisions the particles obey Newtonian rigid body dynamics. All simulation movies and snapshots are generated using VMD software [32] . Details of theoretical development We construct here a hydrodynamic description of the fluid of beads and motile polar rods on a substrate, keeping track of the separately conserved numbers of beads and rods. We show that the flocking transition mediated by the bead velocity is unaltered by the additional conservation law. We demonstrate, in addition, that the presence of the dense fluid of beads leaves unaffected the singular nature [2] of number fluctuations in a flock. This is in contrast to the case [16] of active particles in a confined incompressible fluid medium. Let ρ and σ be the bead and rod concentration fields respectively, and let v be the bead velocity field. Let us identify the polar-rod current with the polar order parameter p as is frequently done in microscopic derivations of the flocking equations [33] . Extending our arguments in the main body of the paper, the governing equations of motion, a two-component extension of the Toner-Tu [2] model, read expressing conservation of beads and polar rods, respectively, which is Newton’s second law for the bead fluid, with damping Γ due to contact with the substrate and lid, propulsion α , and moduli E and F giving rise to pressure-like forces from bead and rod density gradients, and describing the dynamics of the polar order parameter and introducing several phenomenological coefficients. We have ignored two other terms with two factors of p and a single ∇ , which are unimportant to our analysis. The ellipsis in (7) and (8) denotes terms such as ∇ ∇ p , higher orders in p , and [2] order p ∇ p , as well as terms obtained by substituting one or more factors of p in the preceding by v . These include conventional viscous damping ∇ ∇ v . None of these has any significant effect on our analysis. On timescales >> ρ /Γ, (7) tells us that v relaxes to a value determined by the remaining fields. Inserting this value in (6) and (8) yields effective equations of motion for ρ and p , in which (8) retains its form but with a → ā = a − λα /Γ, A → Ā = A + λE /Γ and . For large λα, ā turns negative leading to a flock with mean order parameter p 0 , with magnitude and mean bead velocity v =( α /Γ) p 0 . Let us denote the direction of mean orientation by || and perpendicular directions as ⊥ . Expanding to linear order about this state, p = p 0 +δ p ⊥ , v = v 0 +δ v ⊥ ρ = ρ 0 +δ ρ , σ = σ 0 +δ σ and defining yields for the orientation, with ε 1 = wp 0 , for the concentration of beads, and for the rods. Fourier-transforming in space, and eliminating σ in (10) and (11) via (12) yields and for Fourier components at wavevector q . It is straightforward to see that the eigenfrequencies of this problem are of order q . Using this fact in (13) tells us that q δ ρ q ~Θ q to leading order in q . The term Āq 2 ∂ t δρ q is thus of the same order as the last term . The presence of an additional conserved field, ρ , therefore does not affect the power-counting properties of the equation for the orientational order parameter. If we introduce a noise into (8), the resulting fluctuations in the orientation will scale precisely as in the Toner-Tu flock [2] , and therefore the fluctuations in the concentration of rods, via (12), will be singular. A word on the parameter A : it appears plausible on packing grounds that it should be negative, that is, the thick end of the rod is easier accommodated in low-density regions. However, it proved numerically infeasible to detect density variations on the length scale of a single rod; we defer further discussion of this coefficient to later work as it does not have a significant role in our model. How to cite this article: Kumar, N. et al . Flocking at a distance in active granular matter. Nat. Commun. 5:4688 doi: 10.1038/ncomms5688 (2014).